Generation of folliculogenic human epithelial stem cells from induced pluripotent stem cells Epithelial stem cells (EpSCs) in the hair follicle bulge are required for hair follicle growth and cycling. The isolation and propagation of human EpSCs for tissue engineering purposes remains a challenge. Here we develop a strategy to differentiate human iPSCs (hiPSCs) into CD200 + /ITGA6 + EpSCs that can reconstitute the epithelial components of the hair follicle and interfollicular epidermis. The hiPSC-derived CD200 + /ITGA6 + cells show a similar gene expression signature as EpSCs directly isolated from human hair follicles. Human iPSC-derived CD200 + /ITGA6 + cells are capable of generating all hair follicle lineages including the hair shaft, and the inner and outer root sheaths in skin reconstitution assays. The regenerated hair follicles possess a KRT15 + stem cell population and produce hair shafts expressing hair-specific keratins. These results suggest an approach for generating large numbers of human EpSCs for tissue engineering and new treatments for hair loss, wound healing and other degenerative skin disorders. Induced pluripotent stem cells (iPSCs) have been generated from somatic cells by transduction of reprogramming transcription factors, such as cMYC , SOX2 , KLF4 and OCT4 . The resulting iPSCs resemble embryonic stem cells (ESCs) in their properties and potential to differentiate into a variety of adult cell types. Reprogramming of somatic cells into iPSCs has tremendous potential for clinical application. The pluripotency of iPSCs, along with their genetic identity to specific patients, raises the possibility of their use to treat patients suffering from a myriad of diseases [1] , [2] . However, there remain challenges in differentiating iPSCs into certain cell types. In the skin, epithelial stem cells (EpSCs) in the hair follicle contribute not only to the generation of a new hair follicle with each hair cycle but also to the repair of the epidermis during wound healing [3] , [4] . Hair follicle EpSCs reside in a specialized microenvironment called the bulge, a region at or near the base of the non-cycling portion of each hair follicle [5] . We previously demonstrated that hair follicle EpSCs in human scalp specifically express cytokeratin 15 (KRT15) [6] , [7] , and more recently CD200 and ITGA6 have been shown as surface markers for hEpSCs within hair follicles [8] . The discovery of membrane markers of EpSCs enables researchers to isolate human EpSCs population for functional studies. Human keratinocytes have been reported being derived from ESCs and iPSCs [9] , [10] , [11] . However, directed differentiation of human iPSCs (hiPSCs) or ESCs into folliculogenic EpSCs has not been successful to date and remains an important challenge that needs to be addressed. It is likely that human EpSCs will be useful in the treatment of diseases such as alopecias, ectodermal dysplasias, monilethrix, Netherton syndrome, Menkes disease and hereditary epidermolysis bullosa. Additionally, other skin problems such as burn wounds, chronic wounds and ulcers will benefit from stem cell-related therapies [12] . Here we show that directed differentiation of hiPSCs into EpSCs in vitro can be achieved by precise temporal control of the activities of EGF, retinoic acid (RA) and BMP signalling. The hiPSC-derived EpSCs are sorted based on CD200 and ITGA6 expression. CD200 + /ITGA6 + EpSCs show a similar gene expression signature as that of EpSCs isolated directly from human hair follicles. More importantly, we demonstrate that hiPSC-derived EpSCs reconstitute the epithelial components of the hair follicle and interfollicular epidermis in vivo . Thus, the hiPSC-derived EpSCs are folliculogenic and functionally similar to bulge EpSCs. Generation of hiPSCs from dermal fibroblasts We generated hiPSCs from freshly isolated adult dermal fibroblasts using OCT3/4 , SOX2 and KLF4 as previously described [13] , [14] , [15] , [16] . hiPSC clones exhibiting characteristic human embryonic stem cell (hESC) morphology were isolated ~45 days after transduction ( Supplementary Fig. 1a ). Similar to the H9 hESCs, our hiPSC lines showed high levels of alkaline phosphatase (also known as TRA2-49-6E) activity ( Supplementary Fig. 1b ) and expressed multiple pluripotency markers [14] , [16] , including nuclear transcription factors POU class 5 homeobox 1 (OCT3/4) and nanog homeobox (NANOG) as well as surface antigens SSEA3, SSEA4 and TRA-1-60 ( Supplementary Fig. 1c ). While a series of endogenous stemness genes, including OCT3/4 , NANOG , SRY (sex determining region Y)-box 2 ( SOX2) , REX1 and telomerase reverse transcriptase ( TERT ), were activated in hiPSCs, as revealed by quantitative real-time PCR (qPCR) ( Supplementary Fig. 2 ), and the three retroviral transgenes were silenced ( Supplementary Fig. 3 ). Compared with the parental fibroblasts, hiPSCs displayed extensive demethylation of CpG dinucleotides in the OCT3/4 and NANOG promoters, as shown by bisulphite sequencing ( Supplementary Fig. 4a ). We also found that histone H3 lysine 4 was methylated and histone H3 was acetylated in the promoter regions of OCT3/4 and NANOG in hiPSCs ( Supplementary Fig. 4b ). Pluripotency of the hiPSC clones was confirmed in teratoma formation assays after injection of undifferentiated hiPSCs into immunocompromised NSG mice ( Supplementary Fig. 5 ). Generation of iPSC-derived EpSCs CD200 and ITGA6 are known surface markers for hEpSCs within hair follicles [8] . To generate folliculogenic hEpSCs from hiPSCs, we first followed the prior keratinocyte differentiation protocols [9] , [10] , [11] , [17] . We monitored the temporal expression of CD200 and ITGA6 in differentiating hiPSCs using flow cytometric analysis and found that only a small percentage of cells expressing both CD200 and ITGA6 emerged after 11, 18 of 25 days of differentiation using these protocols ( Fig. 1a,b ). To generate a sufficient number of hEpSCs from hiPSCs, we tried different methods and found that timing of EGF in the culture medium was critical ( Fig. 1b,c and Supplementary Fig. 6 ). Based on these results, we established a new sequential differentiation protocol that used retinoic acid to induce hiPSC to form ectodermal like cells (stage 1), which were then differentiated to form hEpSCs in the presence of BMP4 and EGF (stage 2), followed by the final expansion of the mature keratinocyte lineages in the presence of EGF alone (stage 3, Fig. 2a ). The morphologies of the expected cell types at stages 2 and 3 were shown in Fig. 2b . Using this stage-defined differentiation protocol, we recapitulated the dynamic differentiation process from pluripotent stem cells to EpSCs and then to mature keratinocytes; thus capturing the EpSCs, a transient multipotent stem cell population in vitro . Using the sequential differentiation protocol, the CD200 + /ITGA6 + cells emerged around day 11 after differentiation ( Fig. 2f and Supplementary Fig. 6 ), and reached a maximum level of 26.8±3.0% around day 18 after differentiation ( Fig. 2c,f and Supplementary Fig. 6 ). The appearance of KRT15-positive (KRT15 + ) cells, which reached 29.4%±4.0 by day 18 ( Fig. 1d,g and Supplementary Fig. 7 ), closely paralleled the appearance of the CD200 + /ITGA6 + population. We further analysed the percentage of CD200 + /KRT15 + , CD200 + /keratin 14 (KRT14)-positive (KRT14 + ), KRT15 + /ITGA6 + , KRT14 + /ITGA6 + and KRT15 + /KRT14 + cell populations at day 18. The results demonstrated that these populations did not overlap completely ( Supplementary Fig. 8 ). We analysed the percentage of KRT15 + and ITGB1 + expression among the CD200 + /ITGA6 + cells. Similar to a prior study [18] , we found that only ~50% of CD200 + /ITGA6 + cells expressed KRT15 ( Supplementary Fig. 9 ). As expected from our prior experience with human EpSCs derived from hair follicles, the CD200 + /ITGA6 + population was not stable in culture and their number decreased significantly after day 25 ( Fig. 2f and Supplementary Fig. 6 ); whereas, KRT14 + mature keratinocytes increased steadily over time ( Fig. 2e,h and Supplementary Fig. 10 ), indicating differentiation of hiPSC-derived CD200 + /ITGA6 + cells to more mature keratinocytes. Correspondingly, flow cytometric analysis showed that the pluripotent stem cell (SSEA3 + ) population decreased progressively during differentiation ( Supplementary Fig. 11 ). 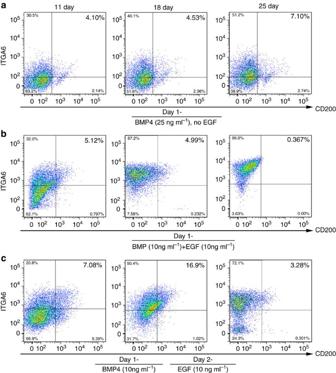Figure 1: Generation of human EpSCs from hiPSCs. (a) Flow cytometric ananlysis of the percentage of CD200+/ITGA6+cell population at day 11, 18 and 25 after hiPSCs were induced with BMP4 and without EGF. (b) Flow cytometric analysis of the percentage of CD200+/ITGA6+cell population at day 11, 18 and 25 after hiPSCs were induced with BMP4 and EGF, while EGF was added 1 day after induction with BMP4. (c) Flow cytometric analysis of the percentage of CD200+/ITGA6+cell population at day 11, 18 and 25 after hiPSCs were induced with BMP4 and EGF, while EGF was added 2 days after induction with BMP4. Figure 1: Generation of human EpSCs from hiPSCs. ( a ) Flow cytometric ananlysis of the percentage of CD200 + /ITGA6 + cell population at day 11, 18 and 25 after hiPSCs were induced with BMP4 and without EGF. ( b ) Flow cytometric analysis of the percentage of CD200 + /ITGA6 + cell population at day 11, 18 and 25 after hiPSCs were induced with BMP4 and EGF, while EGF was added 1 day after induction with BMP4. ( c ) Flow cytometric analysis of the percentage of CD200 + /ITGA6 + cell population at day 11, 18 and 25 after hiPSCs were induced with BMP4 and EGF, while EGF was added 2 days after induction with BMP4. 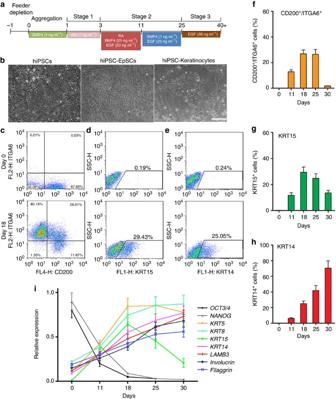Figure 2: Staged differentiation of hiPSCs into human EpSCs. (a) An outline of the protocol used to differentiate hiPSCs to EpSCs and then mature keratinocytes. (b) Morphologies of hiPSCs, hiPSC-derived EpSCs (hiPSC-EpSCs, obtained at day 18 after differentiation) and hiPSC-derived mature keratinocytes (hiPSC-keratinocytes, obtained at day 45 after differentiation). Scale bar, 100 μm. (c–e) Flow cytometric analysis of CD200+/ITGA6+, KRT15+and KRT14+cells at day 0 and 18 during the differentiation. (f–h) Quantification of CD200+/ITGA6+, KRT15+and KRT14+cells by flow cytometric analysis. Data shown are mean±s.d. of cell percentage from three independent experiments. (i) qPCR analysis ofOCT3/4,NANOG,KRT5,KRT8,KRT14,KRT15,LamB3,involucrinandfilaggrinexpression in hiPSC-derived cells at different stages of differentiation. Samples collected at day 0, day 11, day 18, day 25 and day 30 after differentiation were used for qRT–PCR analysis. Data shown are mean±s.d. of the expression from three independent experiments. Full size image Figure 2: Staged differentiation of hiPSCs into human EpSCs. ( a ) An outline of the protocol used to differentiate hiPSCs to EpSCs and then mature keratinocytes. ( b ) Morphologies of hiPSCs, hiPSC-derived EpSCs (hiPSC-EpSCs, obtained at day 18 after differentiation) and hiPSC-derived mature keratinocytes (hiPSC-keratinocytes, obtained at day 45 after differentiation). Scale bar, 100 μm. ( c – e ) Flow cytometric analysis of CD200 + /ITGA6 + , KRT15 + and KRT14 + cells at day 0 and 18 during the differentiation. ( f – h ) Quantification of CD200 + /ITGA6 + , KRT15 + and KRT14 + cells by flow cytometric analysis. Data shown are mean±s.d. of cell percentage from three independent experiments. ( i ) qPCR analysis of OCT3/4 , NANOG , KRT5 , KRT8 , KRT14 , KRT15 , LamB3 , involucrin and filaggrin expression in hiPSC-derived cells at different stages of differentiation. Samples collected at day 0, day 11, day 18, day 25 and day 30 after differentiation were used for qRT–PCR analysis. Data shown are mean±s.d. of the expression from three independent experiments. Full size image We also analysed the temporal gene expression profile of the differentiating cultures and the results demonstrated a step-wise progression from embryonic immature cells ( OCT3/4 + and NANOG + ) to epithelial lineages, characterized by keratin 5 ( KRT5 ) and keratin 8 ( KRT8 ) expression, around 11 days after induction ( Fig. 2i and Supplementary Fig. 12 ). The expression of keratinocyte-specific genes in the differentiating culture derived from hiPSCs increased over time, with concomitant decrease in OCT3/4 and NANOG expression ( Fig. 2i and Supplementary Fig. 12 ). Consistent with flow cytometric analysis results, the expression of KRT15 , began around day 11, peaked around day 18 and then decreased significantly by day 30 ( Fig. 2i and Supplementary Fig. 12 ). Characterization of iPSC-derived EpSCs in vitro EpSCs are known to have high colony-forming efficiency [3] . We compared the colony-forming efficiency of unfractionated cells, CD200 + /ITGA6 + cells, CD200 − /ITGA6 + cells and CD200 + /ITGA6 − cells derived from hiPSCs at day 18 after differentiation; mature keratinocytes were derived from hiPSCs and normal keratinocytes from adult skin as previously described [3] . We found that CD200 + /ITGA6 + cells derived from hiPSCs had the highest colony-forming efficiency among all the epithelial cells, as demonstrated by the higher number and larger size of colonies, compared with the other epithelial cell populations, after 3 weeks in culture ( Fig. 3a and Supplementary Fig. 13 ). Nevertheless, the unfractionated cells formed the most colonies among all the cells tested and hiPSC-derived CD200 + /ITGA6 − cells formed a similar number of colonies to hiPSC-derived CD200 + /ITGA6 + cells ( Supplementary Fig. 13 ). CD200 has been recently reported to be expressed in hiPSCs and hESCs [19] . Our data confirmed the expression of CD200 in hiPSCs, and we found its expression later retained in a subpopulation of ITGA6 + cells as hiPSCs differentiated. Pluripotent stem cell markers, such as OCT3/4 , NANOG and REX1 , were barely detected in cells isolated at day 18 from the CD200 + /ITGA6 + population ( Fig. 3b ), confirming that the hiPSC-derived CD200 + /ITGA6 + cells contain few undifferentiated hiPSCs. However, hiPSC-derived CD200 + /ITGA6 − cells retained expression of ESC markers, including OCT3/4 and NANOG ( Fig. 3b ) with little expression of keratinocyte markers ( Fig. 3c ). The colony morphology formed by CD200 + /ITGA6 − cells was distinctively different from the colony morphology formed by CD200 + /ITGA6 + cells ( Fig. 3d ) and unfractionated cells formed colonies with variable morphologies, supporting that CD200 + /ITGA6 − cells are non-epithelial cells. 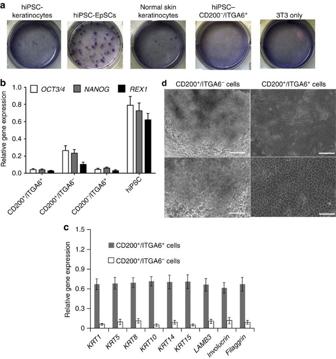Figure 3: Colony formation capacity of hiPSC-derived EpSCs. (a) Colony formation assays. Representative dishes of hiPSC-derived mature keratinocytes (hiPSC-keratinocytes), hiPSC-derived CD200+/ITGA6+cells (hiPSC-EpSCs), passaged normal keratinocytes from adult skin (passage 3) and hiPSC-derived CD200−/ITGA6+cells (hiPSC-CD200−/ITGA6+), cultured for 3 weeks on 3T3 fibroblast feeder cells. The dishes were stained with H&E. Representative images from three independent experiments. (b) qPCR analysis of pluripotent stem cell markers in the hiPSC-derived CD200+/ITGA6+, CD200+/ITGA6−and CD200−/ITGA6+cells. The pluripotent stem cell markers used areOCT3/4,NANOGandREX1. Data shown are mean±s.d. of the expression from three independent experiments. (c) qPCR analysis of the keratinocyte-specific genes in hiPSC-derived CD200+/ITGA6+and CD200+/ITGA6−cells. Data shown are mean±s.d. of the expression from three independent experiments. (d) Morphology of colonies formed by CD200+/ITGA6+and CD200+/ITGA6−cells. Scale bar in upper panel, 100 μm; scale bar in lower panel, 20 μm. Figure 3: Colony formation capacity of hiPSC-derived EpSCs. ( a ) Colony formation assays. Representative dishes of hiPSC-derived mature keratinocytes (hiPSC-keratinocytes), hiPSC-derived CD200 + /ITGA6 + cells (hiPSC-EpSCs), passaged normal keratinocytes from adult skin (passage 3) and hiPSC-derived CD200 − /ITGA6 + cells (hiPSC-CD200 − /ITGA6 + ), cultured for 3 weeks on 3T3 fibroblast feeder cells. The dishes were stained with H&E. Representative images from three independent experiments. ( b ) qPCR analysis of pluripotent stem cell markers in the hiPSC-derived CD200 + /ITGA6 + , CD200 + /ITGA6 − and CD200 − /ITGA6 + cells. The pluripotent stem cell markers used are OCT3/4 , NANOG and REX1 . Data shown are mean±s.d. of the expression from three independent experiments. ( c ) qPCR analysis of the keratinocyte-specific genes in hiPSC-derived CD200 + /ITGA6 + and CD200 + /ITGA6 − cells. Data shown are mean±s.d. of the expression from three independent experiments. ( d ) Morphology of colonies formed by CD200 + /ITGA6 + and CD200 + /ITGA6 − cells. Scale bar in upper panel, 100 μm; scale bar in lower panel, 20 μm. Full size image Next, transcriptional analysis by qPCR showed that EpSC-specific network genes such as LGR5 (ref. 20 ), LGR6 (ref. 21 ), FZD2 , TCF4 , DKK3 , CTNNB1 , LEF1 and LHX2 (ref. 22 ) were activated in CD200 + /ITGA6 + cells derived from hiPSCs and the expression levels were similar to hair follicles EpSCs ( Fig. 4a ). We also analysed these EpSC markers in iPSC-derived KRT14 + /KRT15 + /ITGA6 + cells, and the results showed that the levels of EpSC marker expression in these cells were similar to CD200 + /ITGA6 + cells ( Supplementary Fig. 14 ). Immunocytochemical staining analysis further confirmed the expression of KRT1, KRT10, KRT15 and ITGB1 expression in the hiPSC-derived CD200 + /ITGA6 + cells ( Fig. 4b–e ), respectively; short-term culture of CD200 + /ITGA6 + EpSCs isolated from human hair follicles was used as a control. To further compare the gene expression signature of EpSCs derived from hiPSCs to EpSCs derived from human hair follicles, we analysed global gene expression patterns of CD200 + /ITGA6 + cells isolated from human fetal hair follicles, CD200 + /ITGA6 + cells derived from hiPSCs and the parental hiPSCs. The results showed that hiPSC-derived CD200 + /ITGA6 + cells clustered with CD200 + /ITGA6 + cells isolated from fetal hair follicles, and were distinctively different from the parental hiPSCs as illustrated by unsupervised hierarchical clustering analysis ( Fig. 4f,g ). Notably, there was considerable overlap of genes between hiPSC-derived and hair follicle-derived CD200 + /ITGA6 + cells ( Fig. 4h ), with many representative genes of epithelial lineages, such as KRT1 , KRT8 , KRT10 , KRT15 , ITGB1 and ITGA6 being highly enriched in the CD200 + /ITGA6 + population compared with the parental hiPSCs and their expression levels were similar to EpSCs isolated from human hair follicles ( Supplementary Fig. 15 ). Conversely, expression of the markers of ESCs, such as SOX2 and NANOG , decreased in the hiPSC-derived CD200 + /ITGA6 + cell population ( Fig. 4i ). These findings indicate that the hiPSC-derived CD200 + /ITGA6 + cells share similar molecular signatures with human EpSCs isolated from hair follicles. 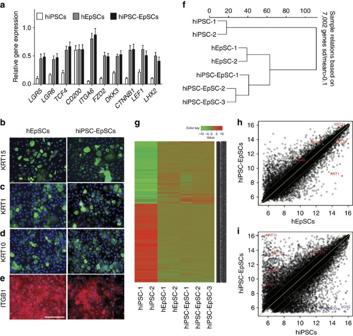Figure 4: Molecular characterization of hiPSC-derived EpSCs. (a) qPCR analysis of known EpSC markers, includingLGR5,LGR6,CD200,KRT15,ITGA6,TCF4,FZD2,DKK3,CTNNB1,LEF1andLHX2in hiPSC-EpSCs compared with control CD200+/ITGA6+cells isolated from fetal hair follicles (hEpSCs) and parental hiPSCs. Data shown are mean±s.d. of the expression from three independent experiments. (b–e) Immunocytochemical analysis of KRT15, KRT1, KRT10 and ITGB1 in hiPSC-EpSCs and hEpSCs culture. Secondary antibodies are conjugated with FITC. Antibody against ITGB1 is conjugated with PE. Scale bar, 50 μm. (f) Hierarchical clustering among the three cell populations analysed. (g) Heat map of genes differentially expressed in RNA-microarray analysis performed on hiPSCs, hiPSC-EpSCs and hEpSCs. (h,i) Scatter plots show that epithelial markers are expressed in hiPSC-EpSCs, whereas iPSCs markers are silenced. Figure 4: Molecular characterization of hiPSC-derived EpSCs. ( a ) qPCR analysis of known EpSC markers, including LGR5 , LGR6 , CD200 , KRT15 , ITGA6 , TCF4 , FZD2 , DKK3 , CTNNB1 , LEF1 and LHX2 in hiPSC-EpSCs compared with control CD200 + /ITGA6 + cells isolated from fetal hair follicles (hEpSCs) and parental hiPSCs. Data shown are mean±s.d. of the expression from three independent experiments. ( b – e ) Immunocytochemical analysis of KRT15, KRT1, KRT10 and ITGB1 in hiPSC-EpSCs and hEpSCs culture. Secondary antibodies are conjugated with FITC. Antibody against ITGB1 is conjugated with PE. Scale bar, 50 μm. ( f ) Hierarchical clustering among the three cell populations analysed. ( g ) Heat map of genes differentially expressed in RNA-microarray analysis performed on hiPSCs, hiPSC-EpSCs and hEpSCs. ( h , i ) Scatter plots show that epithelial markers are expressed in hiPSC-EpSCs, whereas iPSCs markers are silenced. Full size image Characterization of iPSC-derived EpSCs in vivo EpSCs located in the bulge of the hair follicle have been documented to play a crucial role in hair follicle growth and cycling [3] , [5] . Although CD200 and ITGA6 are surface markers for human EpSCs [8] , it is unknown whether human CD200 + /ITGA6 + cells isolated from adult scalp can form hair follicles in skin reconstitution assays. To determine whether hiPSC-derived EpSCs are multipotent and capable of generating all of the epithelial lineages within the skin, we first performed patch assays [23] , [24] for skin reconstitution using day 18 hiPSC-derived CD200 + /ITGA6 + cells, which were enriched by fluorescence-activated cell sorting (FACS) or magnetic bead selection. We found that the magnetic bead approach enabled isolation of large numbers of cells required for in vivo studies with minimal damage to the cells [25] . To minimize contamination of undifferentiated pluripotent stem cells and potential tumorigenesis [26] , [27] , we depleted potential remaining undifferentiated hiPSCs in the CD200 + /ITGA6 + population using magnetic beads conjugated with antibody against the hiPSC membrane marker SSEA3. Neonatal foreskin keratinocytes were used as a positive control, whereas parental hiPSCs, hiPSC-derived CD200 − /ITGA6 + cells at day 18, hiPSC-derived mature keratinocytes or mature keratinocytes isolated from hair bearing normal human skin were used as controls for comparison. The hiPSC-derived CD200 + /ITGA6 + cells or control cells were combined with neonatal mouse dermal cells and injected subcutaneously into the back skin of immune-deficient nude mice. Two and half weeks later the skins of the mice were then excised and examined under a dissecting microscope. Hair follicle-like structures were observed from the underside of the skin ( Fig. 5a and Supplementary Fig. 16 ). Histological analysis revealed that the injected epithelial cells aggregated to form small cystic spheres in the host subcutis. The cysts consisted of both basal keratinocytes and stratified epidermis ( Fig. 5b ). Hair follicles growing outward from the cyst were evident ( Fig. 5b ). This phenomenon was similar to what was observed previously in skin reconstitution assays using mouse EpSCs and neonatal dermal cells [3] , [23] , [24] . We also sorted out CD200 + /ITGA6 + cells from day 11 and 25 cultures and these cells were also capable of forming hair follicles. The human origin of the epithelial cells in the new hair follicle structures and interfollicular epidermis was confirmed by DNA in situ hybridization with a human-specific Alu -repeat sequence probe ( Fig. 5c ). Double DNA in situ hybridization with human and mouse pan-centromeric probes further confirmed that the hair follicle epithelium and interfollicular epidermis were of human origin and the surrounding mesenchymal components were composed of mouse cells ( Fig. 5d,e ). The neonatal foreskin keratinocytes also formed hair follicles and we found that these cells contained distinct populations of CD200 + /ITGA6 + or KRT15 + cells ( Supplementary Fig. 17a ). The qPCR results further confirmed that neonatal foreskin keratinocytes expressed EpSC markers but at a lower level compared with that of hiPSC-derived EpSCs ( Supplementary Fig. 17b ). The other controls including hiPSC-derived mature keratinocytes did not form any hair follicles and flow cytometric analysis showed that few CD200 + /ITGA6 + or KRT15 + cells in the hiPSC-derived mature keratinocytes ( Supplementary Fig. 17a ). These data indicate that EpSCs are required for hair follicle formation. 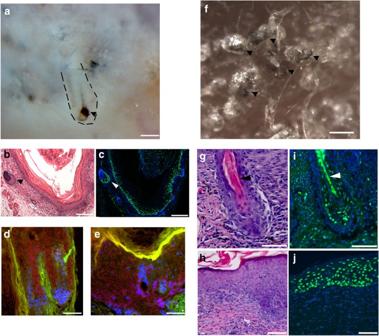Figure 5: Folliculogenic capacity of EpSCs derived from hiPSCs tested in two different types of reconstitution assays. (a) hiPSC-derived CD200+/ITGA6+/SSEA3−cells form hair follicles in a patch reconstitution assay. hiPSC-derived CD200+/ITGA6+/SSEA3−cells were combined with mouse neonatal dermal cells and injected into the dermis of an immunodeficient mouse. After 3 weeks, hair follicles and hair follicle-like structures were observed at the site of injection photographed from the underside of the skin. Dotted short lines outline a hair follicle. An arrowhead points to the pigmented bulb region of a hair follicle. Representative image from seven independent experiments. Scale bar, 500 μm. (b) H&E staining of an epidermal cyst with attached hair follicles formed from hiPSC-EpSCs. An arrowhead points to a hair follicle. Scale bar, 200 μm. (c) Human-specificAluprobe staining (green nuclei) confirms human origin of follicular epithelium and epidermal cyst lining, which were generated by hiPSC-derived EpSCs. An arrowhead points to a hair follicle. Scale bar, 200 μm. (d,e)In situhybridization using pan-centromeric probes specific for human (red) and mouse (green) respectively show human origin of follicular epithelium (d) and epidermal lining (e). Scale bar, 30 μm. (f) Hair follicles form from hiPSC-derived CD200+/ITGA6+/SSEA3−cells and mixed with mouse neonatal dermal cells in a reconstitution assay using a silicone chamber. hiPSC-EpSCs and mouse neonatal dermal fibroblasts were mixed together and placed in a chamber transplanted onto the back skin of a nude mouse29. After 3 weeks, skin and hair follicles formed in the chamber. Pigmented human-like hair shafts were thicker than the surrounding mouse hair shafts. Arrowheads point to the pigmented hair shafts. Scale bar, 1 mm. (g) H&E staining of a reconstituted hair follicle (H&E stain). An arrowhead points to the hair shaft. Scale bar, 150 μm. (h) A human-like multilayered epidermis was formed (H&E stain). Scale bar, 100 μm. (i,j) Human-specificAluprobe staining of human hair follicles (i) and epidermis (j). Human cells were stained by human-specificAluprobe labelled with FITC. An arrowhead points to the hair shaft (i). Scale bar, 150 μm (i), 100 μm (j). Representative images from three independent experiments. Figure 5: Folliculogenic capacity of EpSCs derived from hiPSCs tested in two different types of reconstitution assays. ( a ) hiPSC-derived CD200 + /ITGA6 + /SSEA3 − cells form hair follicles in a patch reconstitution assay. hiPSC-derived CD200 + /ITGA6 + /SSEA3 − cells were combined with mouse neonatal dermal cells and injected into the dermis of an immunodeficient mouse. After 3 weeks, hair follicles and hair follicle-like structures were observed at the site of injection photographed from the underside of the skin. Dotted short lines outline a hair follicle. An arrowhead points to the pigmented bulb region of a hair follicle. Representative image from seven independent experiments. Scale bar, 500 μm. ( b ) H&E staining of an epidermal cyst with attached hair follicles formed from hiPSC-EpSCs. An arrowhead points to a hair follicle. Scale bar, 200 μm. ( c ) Human-specific Alu probe staining (green nuclei) confirms human origin of follicular epithelium and epidermal cyst lining, which were generated by hiPSC-derived EpSCs. An arrowhead points to a hair follicle. Scale bar, 200 μm. ( d , e ) In situ hybridization using pan-centromeric probes specific for human (red) and mouse (green) respectively show human origin of follicular epithelium ( d ) and epidermal lining ( e ). Scale bar, 30 μm. ( f ) Hair follicles form from hiPSC-derived CD200 + /ITGA6 + /SSEA3 − cells and mixed with mouse neonatal dermal cells in a reconstitution assay using a silicone chamber. hiPSC-EpSCs and mouse neonatal dermal fibroblasts were mixed together and placed in a chamber transplanted onto the back skin of a nude mouse [29] . After 3 weeks, skin and hair follicles formed in the chamber. Pigmented human-like hair shafts were thicker than the surrounding mouse hair shafts. Arrowheads point to the pigmented hair shafts. Scale bar, 1 mm. ( g ) H&E staining of a reconstituted hair follicle (H&E stain). An arrowhead points to the hair shaft. Scale bar, 150 μm. ( h ) A human-like multilayered epidermis was formed (H&E stain). Scale bar, 100 μm. ( i , j ) Human-specific Alu probe staining of human hair follicles ( i ) and epidermis ( j ). Human cells were stained by human-specific Alu probe labelled with FITC. An arrowhead points to the hair shaft ( i ). Scale bar, 150 μm ( i ), 100 μm ( j ). Representative images from three independent experiments. Full size image To further confirm the folliculogenic capacity of hiPSCs-derived EpSCs, we performed a chamber-based skin reconstitution assay [28] , [29] using hiPSC-derived EpSCs and neonatal mouse dermal cells. The hiPSC-derived EpSCs were mixed with C57BL/6 neonatal dermal fibroblasts in a chamber and transplanted onto mouse back skin. Three weeks later hair follicle-like structures were observed in the grafts ( Fig. 5f and Supplementary Fig. 16 ). Histological examination showed large human-like hair follicles with hair shafts, which were distinctively different from mouse hair shafts in the grafts ( Fig. 5f,g ). Human-like multilayered epidermis was also formed in the grafts ( Fig. 5h ). The newly formed epidermis was impermeable to toluidine blue dye, indicating a functional skin barrier ( Supplementary Fig. 18 ). Human origin of the epithelial cells in the hair follicles and epidermis was confirmed by DNA in situ hybridization with a human-specific Alu -repeat sequence probe ( Fig. 5i,j ). Next, we performed immunostaining to characterize the hair follicles and epidermis originating from hiPSC-derived EpSCs. We found that KRT15 was expressed in the bulge region of the chimeric hair follicles ( Fig. 6a , right panel), similar to hair follicles formed by neonatal foreskin keratinocytes ( Fig. 6a , left panel). Other keratinocyte markers, such as KRT14, were detected in the outer root sheath of the chimeric hair follicles ( Fig. 6b ). H&E staining showed that the innermost regions of the chimeric hair follicle structures resembled the hair cortex and the medulla of mature human hair follicles ( Fig. 6c–e ). The formation of such structures were further confirmed by immunohistochemical staining for AE13, a marker for hair follicle cortex, and AE15, a marker for inner root sheath and medulla, in a pattern that is similar to normal human hair follicles ( Fig. 6c,d and Supplementary Fig. 19a,b ). We also found K75 expressed specifically in the companion layer of the chimeric hair follicle ( Fig. 6e and Supplementary Fig. 19c ). The hiPSC-derived CD200 + /ITGA6 + cells not only reconstituted the epithelial components of the hair follicle but also the interfollicular epidermis. The multilayered interfollicular epidermis expressed KRT10 and involucrin ( Fig. 6f,g ). Our findings indicate that hiPSC-derived CD200 + /ITGA6 + cells are capable of generating functional epidermis and they respond to inductive dermal signals to generate the epithelial component of hair follicles. 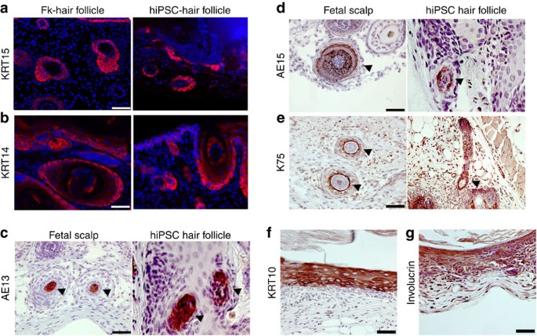Figure 6: Characterization of hair follicles and interfollicular epidermis formed by hiPSC-EpSCs. (a,b) Reconstitution of stem cell niche in hair follicles by EpSCs derived from hiPSCs. CD200+/ITGA6+/SSEA3−cells derived from hiPSCs were combined with mouse neonatal dermal cells and injected into the dermis of an immunodeficient mouse. Neonatal foreskin keratinocytes (Fk) were used as a positive control. Immunostaining of reconstituted hair follicles formed by neonatal foreskin keratinocytes or hiPSC-EpSCs was performed using antibodies against KRT15 (a) or KRT14 (b), respectively. Scale bar, 100 μm. hiPSC-hair follicle represents the hair follicle derived from hiPSC-EpSCs. FK hair follicle represents the hair follicle formed by neonatal foreskin keratinocytes. (c–e) Immunostaining of hair follicles formed by hiPSC-EpSCs using hair differentiation markers AE13 (c), AE15 (d) and K75 (e). Arrowheads point to the positive areas. Fetal scalp tissue was sectioned and stained with antibodies against AE13, AE15 and K75, respectively as positive controls. AE13 marks hair follicle cortex and AE15 marks inner root sheath and medulla. K75 marks companion layer of a hair follicle. Scale bar, 100 μm. (f,g) Immunostaining of interfollicular epidermal lining of cyst formed by hiPSC-EpSCs was performed using antibodies against KRT10 (f) or Involucrin (g). Scale bar, 50 μm. Figure 6: Characterization of hair follicles and interfollicular epidermis formed by hiPSC-EpSCs. ( a , b ) Reconstitution of stem cell niche in hair follicles by EpSCs derived from hiPSCs. CD200 + /ITGA6 + /SSEA3 − cells derived from hiPSCs were combined with mouse neonatal dermal cells and injected into the dermis of an immunodeficient mouse. Neonatal foreskin keratinocytes (Fk) were used as a positive control. Immunostaining of reconstituted hair follicles formed by neonatal foreskin keratinocytes or hiPSC-EpSCs was performed using antibodies against KRT15 ( a ) or KRT14 ( b ), respectively. Scale bar, 100 μm. hiPSC-hair follicle represents the hair follicle derived from hiPSC-EpSCs. FK hair follicle represents the hair follicle formed by neonatal foreskin keratinocytes. ( c – e ) Immunostaining of hair follicles formed by hiPSC-EpSCs using hair differentiation markers AE13 ( c ), AE15 ( d ) and K75 ( e ). Arrowheads point to the positive areas. Fetal scalp tissue was sectioned and stained with antibodies against AE13, AE15 and K75, respectively as positive controls. AE13 marks hair follicle cortex and AE15 marks inner root sheath and medulla. K75 marks companion layer of a hair follicle. Scale bar, 100 μm. ( f , g ) Immunostaining of interfollicular epidermal lining of cyst formed by hiPSC-EpSCs was performed using antibodies against KRT10 ( f ) or Involucrin ( g ). Scale bar, 50 μm. Full size image Sebocytes and mature keratinocytes from iPSC-derived EpSCs To further define the differentiation capacity of hiPSC-derived CD200 + /ITGA6 + cells, we cultured these cells under sebocyte differentiation conditions as previous described [30] . Three weeks after differentiation, some of the cells acquired abundant cytoplasm with oil droplets that were positive for oil red staining ( Supplementary Fig. 20a ). The sebocyte-like cells also expressed sebocyte markers, such as keratin 7 ( KRT 7 ), peroxisome proliferator-activated receptor alpha ( PPAR-α or PPARA ) and lipoprotein lipase ( LPL ), as shown by qPCR ( Supplementary Fig. 20b ). To the contrary, hiPSC-derived mature keratinocytes could not be differentiated into sebocytes under the same condition. These results indicate that hiPSC-derived CD200 + /ITGA6 + cells are capable of sebocyte differentiation. In order to generate mature keratinocytes from hiPSC-derived CD200 + /ITGA6 + cells, the hiPSC-derived EpSCs were cultured for an additional 25 days in the presence of EGF until the KRT14 + keratinocytes population reached 98.8% purity as shown by flow cytometric analysis, whereas CD200 + /ITGA6 − cells cultured under the same conditions resulted in generating only 18.0% KRT14 + keratinocytes ( Fig. 7a ). Transcriptional analysis by qPCR showed that KRT14 + keratinocytes derived from hiPSC expressed a panel of epidermal genes similar to those of normal skin keratinocytes ( Fig. 7b ). Immunostaining analysis showed that most cells expressed mature squamous cell markers, such as keratin proteins (KRT14), p63, integrins (ITGA6 and ITGB4), pan-cytokeratin and E-cadherin (also known as CDH1) ( Fig. 7c–g ). We next generated 3D skin equivalents using keratinocytes from foreskin and mature keratinocytes from hiPSC-derived CD200 + /ITGA6 + cells. The 3D skin equivalents exhibited a multilayered epidermis, expressing squamous differentiation markers such as KRT14 and KRT5, and also epithelial markers Pan-cytokeratin (Pan-CK) ( Fig. 7h ), in a pattern similar to skin equivalents formed by foreskin keratinocytes. These data support that hiPSC-derived CD200 + /ITGA6 + cells are multipotent. However, surprisingly, we were not able to identify human sebaceous glands derived from the hiPSC-derived CD200 + /ITGA6 + cells or neonatal foreskin keratinocytes in the skin reconstitution assays. It is well known that mouse EpSCs (CD34 + /ITGA6 + or KRT15 high /ITGA6 + ) are capable of regenerating both follicular epithelium and sebaceous units in the skin reconstitute assays [3] , [31] . These results suggest that hiPSC-derived CD200 + /ITGA6 + cells, although folliculogenic and sharing molecular signatures similar to those of human EpSCs, are likely more restricted in their lineage potential compared with EpSCs or they may require additional signals for sebocyte differentiation in vivo . 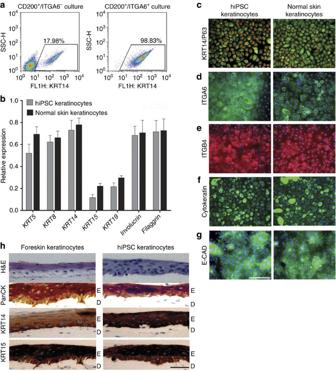Figure 7: Differentiation of hiPSCs into mature keratinocytes. (a) Flow cytometric analysis of the hiPSC-derived mature keratinocytes. hiPSC-derived CD200+/ITGA6+and CD200−/ITGA6+cells were cultured for additional 25 days and flow cytometric analysis was performed to detect the number of KRT14+cells. (b) qPCR analysis of keratinocyte markers. Keratinocyte markers, includingKRT5,KRT8,KRT14,KRT15,KRT19,InvolucrinandFilaggrin, were analysed by qPCR in mature keratinocytes derived from hiPSCs (hiPSC-keratinocytes) and normal skin-derived keratinocytes (normal skin keratinocytes). Data shown are mean±s.d. of the expression from three independent experiments. (c–g) Immunocytochemical stains of keratinocytes markers, including KRT14, p63, ITGA6, pan-cytokeratin, ITGB4 and E-cadherin (E-CAD) in hiPSC-derived mature keratinocytes (hiPSC-keratinocytes) and normal skin keratinocytes, Scale bar, 20 μm. (h) 3D skin equivalents using hiPSC-derived mature keratinocytes. Neonatal foreskin-derived keratinocytes (foreskin keratinocytes) were used as a control. H&E stain of the 3D skin equivalents showed multilayered epidermis. The epidermis expressed pan-cytokeratin (Pan-CK), KRT5 and KRT14. Scale bar, 30 μm. Figure 7: Differentiation of hiPSCs into mature keratinocytes. ( a ) Flow cytometric analysis of the hiPSC-derived mature keratinocytes. hiPSC-derived CD200 + /ITGA6 + and CD200 − /ITGA6 + cells were cultured for additional 25 days and flow cytometric analysis was performed to detect the number of KRT14 + cells. ( b ) qPCR analysis of keratinocyte markers. Keratinocyte markers, including KRT5 , KRT8 , KRT14 , KRT15 , KRT19 , Involucrin and Filaggrin , were analysed by qPCR in mature keratinocytes derived from hiPSCs (hiPSC-keratinocytes) and normal skin-derived keratinocytes (normal skin keratinocytes). Data shown are mean±s.d. of the expression from three independent experiments. ( c – g ) Immunocytochemical stains of keratinocytes markers, including KRT14, p63, ITGA6, pan-cytokeratin, ITGB4 and E-cadherin (E-CAD) in hiPSC-derived mature keratinocytes (hiPSC-keratinocytes) and normal skin keratinocytes, Scale bar, 20 μm. ( h ) 3D skin equivalents using hiPSC-derived mature keratinocytes. Neonatal foreskin-derived keratinocytes (foreskin keratinocytes) were used as a control. H&E stain of the 3D skin equivalents showed multilayered epidermis. The epidermis expressed pan-cytokeratin (Pan-CK), KRT5 and KRT14. Scale bar, 30 μm. Full size image In this study, we present a method to differentiate hiPSCs into functional EpSCs that are capable of reconstituting the epithelial components of the hair follicle and interfollicular epidermis in the skin regeneration assays. Since human hair follicle cycling lasts for years, it is not possible to study human hair follicle cycling using the xenograft models, and thus it is difficult to assess the long-term renewal of the transplanted hiPSC-derived EpSCs. It is interesting that at day 18 after differentiation, numbers of Lrig1 + /ITGA6 + cells, Lrg6 + /ITGA6 + cells or MTS24 + /ITGA6 + cells are also present in the culture ( Supplementary Fig. 21 ). Although the function of these human cell populations is unknown, the different epidermal lineages after CD200 + /ITGA6 + cells grafting may arise from multipotent stem cell population and potentially different unipotent stem cell populations. Previous study demonstrated that mouse iPSC-derived multipotent keratinocytes induced by BMP4 can reconstitute normal skin and its appendages in an in vivo assay [32] . Veraitch et al. [33] used a similar protocol and they found that the hiPSC-derived ectodermal precursor cells emerging at day 11 contributed to hair follicle morphogenesis. However, it was unclear from the study which cell population in the ectodermal cells contributed to folliculogenesis, and the hair shaft shown in the study appeared to be of mouse origin. The authors suggest that low frequency of human-derived cells in the hair follicles observed in their study implied that these cells contribute to hair follicle morphogenesis via direct repopulation and non-cell autonomous activities [33] . We observed only small percentage of CD200 + /ITGA6 + cells at day 11 when we tested a similar protocol without using EGF, and >30% of the cells retained expression of SSEA3 ( Supplementary Fig. 22 ), which are undifferentiated and potentially tumorigenic iPSCs. We depleted SSEA3 + cells before in vivo reconstitution assays. More importantly, hiPSC-derived EpSCs are capable of re-establishing the hair follicle bulge region with KRT15 + cells in our work. In conclusion, we developed a novel hiPSC differentiation method that efficiently differentiates hiPSCs to EpSCs, and these CD200 + /ITGA6 + cells have similar molecular characteristics of hEpSCs. The hiPSC-derived CD200 + /ITGA6 + cells isolated by magnetic beads provide a simple approach for generating highly enriched populations of folliculogenic human cells that can reconstitute the hair follicle epithelial components and interfollicular epidermis in vivo . Our study establishes a means for obtaining a scalable source of human EpSCs, which is a major step toward developing cell-based treatments for hair loss and other skin disorders. However, the current protocol to obtain hiPSC-derived EpSCs is not FDA-friendly and will need to be thoroughly validated. Nevertheless, access to cells with cardinal features of hEpSCs opens new possibilities for studying regenerative therapies for hair loss, wound healing and ageing skin. Cell culture Human primary fibroblasts were obtained from discarded normal skin after surgery following a protocol approved by the University of Pennsylvania Institutional Review Board. HEK 293T cells and human fibroblasts were cultured in DMEM supplemented with 10% fetal bovine serum (FBS), 2 mM L -glutamine, 100 unit per ml penicillin and 100 μg per ml of streptomycin (all from Invitrogen). The hiPSCs were cultured on MEF feeders using hESC culture medium that contains 80% DMEM/F12 (1:1) medium, 20% knockout Serum Replacement, 100 μM non-essential amino acids, 2 mM L -glutamine, 0.1 mM β-mercaptoethanol, 100 unit per ml penicillin, 100 μg per ml streptomycin and 10–15 ngper ml bFGF (all from Invitrogen). hiPSC generation with retroviral infection To prepare the retroviruses, HEK 293T cells were transfected with pMXs plasmids containing the coding sequences for SOX2 , OCT3/4 , and KLF4 , along with pUMVC and pCMV-VSV-G plasmids at the ratio of 10 μg of plasmid DNA to 20 μl of Fugene 6 (Roche) in 500 μl Opi-MEM (Invitrogen). The ratio of pMXs:pUMVC:pCMV-VSV-G was 3:2:1. Next day, the culture medium containing the retroviruses was harvested and concentrated by Retro-X Concentrator (TAKARA). The human fibroblasts were plated at 1 × 10 5 cells per well in the six-well plate 1 day before infecting with the retroviruses. The retrovirus solution was added to the fibroblasts and incubated overnight. Twenty four hours after the infection, infected fibroblasts were plated in gelatin-coated 100-mm dishes containing irradiated feeder cells. One day after plating on feeder cells, the medium was changed to hESC culture medium. hESC-like clones were observed 25–30 days after the initial infection. The hiPSC clones were picked up ~45 days after the initial infection. Eight lines of hiPSC were established from eight different donors and used in the subsequent experiments. Characterization of hiPSCs We performed reverse transcription reactions using SuperScript III First-Strand Synthesis kit (Invitrogen). PCR was done with PCR Master Mix (Promega). The primer sets used for RT–PCR are listed in Supplementary Table 1 . Alkaline phosphatase detection kit (Sigma) was used to detect alkaline phosphatase activity. Bisulphite genomic sequencing was performed using the CpGenome modification kit (Millipore) according to the manufacturer’s recommendations. Amplified products were cloned into pCR2.1-TOPO (Invitrogen). Ten randomly selected colonies were sequenced with the M13 forward and M13 reverse primers for each gene [14] , [16] , [34] . Sequencing was performed at the University of Pennsylvania sequencing facility. For histone modification, 10 7 hiPSCs, hESCs or hFs were fixed with 1% formaldehyde for 10 min and then lysed in 1 ml lysis buffer (50 mM Tris–HCl, pH 8.0, 10 mM EDTA, 1% SDS, and protease inhibitors) for 20 min on ice. The lysate was split into three tubes and sonicated. After 10 min centrifugation, the supernatant was pre-cleared for 4 h at 4 °C with agarose beads and normal IgG in IP buffer (50 mM Tris–HCl (pH 8.0), 150 mM NaCl, 2 mM EDTA, 1% NP-40, 0.5% sodium deoxycholate, 0.1% SDS and protease inhibitors). A total of 100 ul of pre-cleared chromatin per reaction diluted in 1 ml IP buffer in the presence of 20 ug antibody was used for each immunoprecipitation reaction according to the manufacturer’s protocol. The antibodies used for this study were anti-acH3 (Millipore), anti-dimethyl K4 of H3 (Millipore) and normal rabbit IgG (Sigma). The precipitate was purified and analysed by qPCR using Bio Rad SYBR Green qPCR Master Mix [14] , [16] , [34] . For teratoma formation, 10 6 hiPSCs were injected into the flank of NSG mice (The Jackson Laboratory). The tumours were examined histologically for the presence of different lineages of cells. Differentiation of hiPSCs into CD200 + /ITGA6 + cells and keratinocytes Prior to differentiation, the cells were feeder-depleted by culturing on a thin layer of matrigel (BD Biosciences) in hESC medium for 24 to 48 h. For differentiation, cells were dissociated to small clusters (10–20 cells) with collagenase IV (1 mg ml −1 , Invitrogen) for 20 min followed by trypsin-EDTA (0.05%) for ~2 min. The clusters were washed and cultured in the six-well low-cluster plate (Corning) in 2 ml hESC medium containing Y27632 without bFGF to form embryoid bodies. Embryoid bodies were seeded onto mitomycin-C-treated 3T3 fibroblasts in differentiation medium. Cells were grown in the differentiation medium until clones of epithelial cells were observed and isolated around day 11. The epithelial cells were plated and cultured on 3T3 fibroblasts again until the population of CD200 + /ITGA6 + cells reached their maximum level around day 18. The CD200 + /ITGA6 + cells were sorted out and cultured in the differentiation medium containing EGF. The characteristic mature keratinocytes were obtained by day 40 after the differentiation. For differentiation to the epithelial lineage, the following molecules were used: days 0–1, BMP4 (1 ng ml −1 , R&D system); days 1–11, all-trans RA (1 μM, Sigma-Aldrich); days 3–11, BMP4 (25 ng ml −1 ), EGF (20 ng ml −1 , R&D system); days 11–25, BMP4 (1 ng ml −1 ), EGF (20 ng ml −1 ); days 25 and after, EGF (20 ng ml −1 ). Initiation medium (3:1 mixture of DMEM and Ham’s F12 medium with 2% FBS, 5 μg ml −1 insulin, 0.5 μg ml −1 hydrocortisone, 10 −10 mol l −1 cholera toxin, 1.37 ng ml −1 triiodothyronine, 0.3 mmol l −1 L -ascorbic acid and 24 μg ml −1 adenine) was used at day 1–7. Induced medium 1 (Defined Keratinocyte-SFM (Invitrogen) with 5 μg ml −1 insulin, 0.2 μg ml −1 hydrocortisone, 10 −10 mol l −1 cholera toxin, 1.37 ng ml −1 triiodothyronine, 0.3 mmol l −1 L -ascorbic and 10 μg ml −1 adenine) was used at day 8–11. Induced medium 2 (1:1 mixture of Keratinocyte-SFM (Invitrogen) and Defined Keratinocyte-SFM) was used at day 11–25. Induced medium 3 (Keratinocyte-SFM) was used after day 25. Flow cytometry and cell sorting Cells were stained at a concentration of 2.5 × 10 6 cells per ml with antibodies against CD200, ITGA6, SSEA3, KRT14 and KRT15. For cell-surface markers, staining was carried out in PBS with 2% FBS. For intracellular proteins, staining was carried out on cells fixed with 4% paraformaldehyde (Electron Microscopy Sciences) in PBS. Staining was done in PBS with 2% FBS. Stained cells were analysed using an LSRII flow cytometer (BD Biosciences). For FACS, the cells were sorted at a concentration of 10 6 cells per ml in PBS/2% FBS using a FACS AriaTMII cell sorter (BD Biosciences). For magnetic bead sorting, the Miltenyi MACS bead sorting system was used according to the manufacturer’s guidelines and sorting conditions. Data were analysed using FlowJo software (Treestar). A comprehensive list of antibodies is described in Supplementary Table 2 . Patch assay for skin reconstitution hiPSC-derived CD200 + /ITGA6 + /SSEA3 − cells were isolated and combined with freshly isolated dermal cells from neonatal mice. In all experiments, approximately equal numbers of epithelial and dermal cells (1 million each) were combined at a concentration of 10 4 cells per μl in DMEM/F12 and injected subcutaneously into immune-compromised NU/NU nude mouse. The animal protocol has been approved by the University of Pennsylvania Institutional Animal Care and Use Committee. Two and a half weeks after implantation, the mice were killed and the subcutaneous growths were dissected and processed for histology and immunohistochemistry analysis. A comprehensive list of antibodies is provided in Supplementary Table 2 . Appropriate Alexa488 or Alexa590 -conjugated secondary antibodies (Molecular Probes) were used with 4′,6-diamidino-2-phenylindole (DAPI) nuclear counterstain (Vector lab). Patch assays using hiPSC-EpSCs and various controls were repeated independently for seven times in 20 mice. Chamber assay for skin reconstitution The cellular grafting procedure for hair follicle reconstitution in vivo was performed [28] , [29] , [35] . Briefly, hiPSC-derived EpSCs and mouse neonatal dermal cells (5 million each) were resuspended individually or mixed together in the medium and were then transferred to grafting chambers implanted on the back skins of immune-compromised NU/NU Nude mouse. The chambers were removed 1 week after grafting, and hair follicle formation was assessed at 3–4 weeks. Part of each grafting site was dissected for histological observation. The assays were repeated three times. Skin permeability assay The reconstituted skin were rinsed in PBS and immersed in methanol successively; they were then rehydrated in PBS and stained in 0.1% toluidine blue, which was resolved in H 2 O or DMSO for 10 min at room temperature. They were briefly washed in PBS and were immediately photographed. Global gene profiling and array analysis RNA from hiPSCs, hEpSCs and hiPSCs-EpSCs was isolated. Profiling study was performed using human whole-genome expression chips (Illumina) at the Wistar Institute microarray core. Microarray raw data generated from Illumina Chip were normalized, background-corrected and summarized using the R package ‘lumi’ [36] . To reduce false positives, the unexpressed probes were removed, leaving 21,758 probes that were examined in all experiments described herein. The R package ‘limma’ [37] , [38] was employed for gene differentially expression analysis, followed by multiple test correction by the Benjamini and Hochberg procedure [39] . The genes with the adjusted P -values <0.05 and fold change >4 were subjected to two-way clustering analysis for generating the heat map. In situ hybridization Briefly, paraffin slides were dehydrated, antigen retrieved and hybridized with Alu DNA probe (BioGenex); the slide was heated to 85 °C for 10 min and then 37 °C overnight. The slides were then incubated with antibody specific for fluorescein, biotin-labelled (BioGenex) and finally incubated with secondary antibody labelled with Streptavidin–Alexa Fluo488. DAPI was used to label the nuclear DNA. Statistical analysis Student’s t- test or ANOVA was used to analyse gene expression and flow cytometric data. qPCR data were analysed after being normalized for β-actin loading control. Statistical significance was determined if two-sided P <0.05. Accession Codes : Microarray data has been deposited in Gene Expression Omnibus under accession number GSE51028 . How to cite this article: Yang, R. et al. Generation of folliculogenic human epithelial stem cells from induced pluripotent stem cells. Nat. Comm. 5:3071 doi: 10.1038/ncomms4071 (2014).